Evolutionarily conserved intracellular gate of voltage-dependent sodium channels Members of the voltage-gated ion channel superfamily (VGIC) regulate ion flux and generate electrical signals in excitable cells by opening and closing pore gates. The location of the gate in voltage-gated sodium channels, a founding member of this superfamily, remains unresolved. Here we explore the chemical modification rates of introduced cysteines along the S6 helix of domain IV in an inactivation-removed background. We find that state-dependent accessibility is demarcated by an S6 hydrophobic residue; substituted cysteines above this site are not modified by charged thiol reagents when the channel is closed. These accessibilities are consistent with those inferred from open- and closed-state structures of prokaryotic sodium channels. Our findings suggest that an intracellular gate composed of a ring of hydrophobic residues is not only responsible for regulating access to the pore of sodium channels, but is also a conserved feature within canonical members of the VGIC superfamily. Voltage-gated sodium channels are transmembrane proteins critical for initiation and propagation of electrical signals in a variety of excitable cells [1] . In response to membrane depolarization, these channels open to allow ion flux, contributing to the rising phase of an action potential [2] . Voltage sensitivity is conferred by four discrete voltage-sensing domains connected to the gates in the pore domain of the sodium channel [3] . This basic architecture is conserved among members of the voltage-gated ion channel (VGIC) superfamily, one of the largest families of signalling proteins [4] . Despite their overall similarity, it is becoming clear with the advent of new structures that there are significant structural differences amongst the members of this superfamily that contribute to their functional diversity [5] , [6] , [7] , [8] , [9] . In the case of eukaryotic voltage-gated sodium channels, a founding member of the VGIC superfamily, the molecular features that underpin the moving parts of the pore gate remain unclear. Accessibility studies on the Shaker potassium channel revealed that an intracellular gate comprised of the cytoplasmic ends of the S6 helices controls ion access to the pore [10] , [11] . Similarly, permeation in a voltage-gated calcium channel was shown to be regulated by an intracellular gate [12] . In contrast, accessibility studies on cyclic nucleotide-gated (CNG) channels have shown that a pore gate is formed not by the S6 helices, but at the extracellular selectivity filter [13] , [14] . For the calcium- and voltage-gated (BK) channels, the pattern of accessibility shows that residues all the way up to the selectivity filter remain partially accessible even when the channel is closed, consistent with a gate at the selectivity filter similar to CNG channels [5] , [15] . The above findings raise a number of related questions about the location of the pore gate in this superfamily. First, where is the activation gate in a voltage-gated sodium channel? Second, if this gating is not a conserved feature, what makes it different? Finally, is structural data compatible with cysteine accessibility measurements? Recently, structures of distantly related bacterial sodium channels in closed and putative open states suggest that the intracellular bundle crossing formed by the S6 helices may gate the access of ions into the pore [8] , [16] , [17] , [18] . Substituted cysteine accessibility measurements on voltage-gated sodium channels have been hampered by fast inactivation, which reflects a rapid occlusion of the pore by an inactivation particle during channel activation [19] . This secondary gate complicates accessibility studies because intracellularly applied reagents cannot access the pore when it is obstructed by the inactivation gating motif. Indeed, accessibility studies of other channels were performed in the absence of fast inactivation [5] , [10] , [13] . Until now, this was not possible in sodium channels because the mutations that removed fast inactivation severely compromised channel expression [20] . Recently, we and others have characterized a different inactivation-deficient mutant (WCW) which expresses robust currents, making this system amenable for detailed biophysical studies [21] , [22] . Here we assay the state-dependent accessibility of substituted cysteines in domain IV S6 in this fast inactivation-removed background to test the hypothesis that the pore gate in a voltage-gated sodium channel is located intracellularly. We observe a clear separation of state-dependent accessibility with respect to position along the DIV S6 helix, with positions I1589 and below (extracellular side) having 10,000-fold or greater changes in accessibility between closed and open states, whereas positions I1590 and below (intracellular) are accessible even when the channel are closed. Sequence analysis shows that this transition in accessibility occurs within a hydrophobic region that is highly conserved within canonical members of the VGIC superfamily. Furthermore, our accessibility data are compatible with the structural data derived from closed- and open-state structures of prokaryotic sodium channels that support the notion that prokaryotic sodium channels may serve as good model systems to study pore gating of eukaryotic sodium channels under certain circumstances. Nav1.4-WSW as a background for MTSET accessibility studies To probe the pore of a voltage-gated sodium channel with thiol-modifying reagents such as 2-(trimethylammonium)ethyl methanethiosulfonate (MTSET), it is necessary to use a mutant channel that does not fast inactivate and does not contain any endogenous cysteines that can react with MTSET. We have previously demonstrated that Nav1.4-WCW (L435W/L437C/A438W) almost completely removes fast inactivation while preserving wild-type activation properties at a single channel level [22] . Nav1.4-WCW, however, can be modified by MTSET [22] . To overcome this problem, we generated Nav1.4-WSW (L435W/L437S/A438W) and established that this mutant has macroscopic behaviour similar to Nav1.4-WCW in that it lacks fast inactivation [22] . To determine whether this mutant can be modified by MTSET, sodium currents were monitored after repeated applications of 800 μM MTSET to the intracellular surface of inside-out patches containing Nav1.4-WSW channels while they were either closed or open. Peak sodium currents did not decline after each exposure period, indicating that Nav1.4-WSW does not react with MTSET in either closed or open states ( Fig. 1a,b ). These results demonstrate that Nav1.4-WSW can be used as a background for experiments involving cysteine-reactive chemicals. 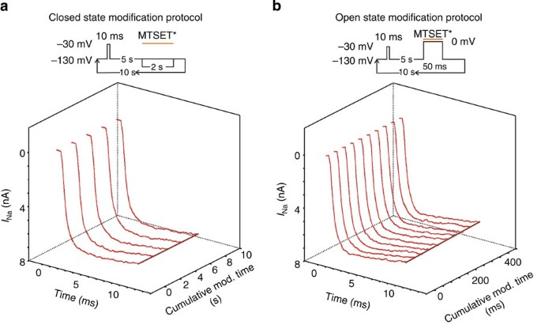Figure 1: Establishment of Nav1.4-WSW as a suitable background for MTSET accessibility studies. Closed-state (a, top) and open-state (b, top) modification protocols for monitoring modification by 800 μM MTSET applied to inside-out patches excised fromXenopusoocytes containing Nav1.4-WSW channels. For the closed-state modification protocol, channels were held at −130 mV, given a 10-ms test pulse to −30 mV, and then subjected to two seconds of MTSET treatment at −130 mV (orange bar indicates the duration of MTSET perfusion). This process was repeated every 10 s with MTSET washout occurring at −130 mV. Test pulse current traces are plotted before and after each subsequent exposure to MTSET (a, bottom). For the open-state modification protocol, channels were held at −130 mV, given a 10-ms test pulse to −30 mV, and then exposed to MTSET for 50 ms at 0 mV. This process was repeated every 40 s with MTSET washout occurring at −130 mV. Test pulse current traces are plotted before and after each subsequent exposure to MTSET (b, bottom). The brown line was included to highlight any changes in current amplitude. Peak sodium current does not decrease after exposure to MTSET while channels are closed or open, indicating that this mutant does not react with MTSET. Figure 1: Establishment of Nav1.4-WSW as a suitable background for MTSET accessibility studies. Closed-state ( a , top) and open-state ( b , top) modification protocols for monitoring modification by 800 μM MTSET applied to inside-out patches excised from Xenopus oocytes containing Nav1.4-WSW channels. For the closed-state modification protocol, channels were held at −130 mV, given a 10-ms test pulse to −30 mV, and then subjected to two seconds of MTSET treatment at −130 mV (orange bar indicates the duration of MTSET perfusion). This process was repeated every 10 s with MTSET washout occurring at −130 mV. Test pulse current traces are plotted before and after each subsequent exposure to MTSET ( a , bottom). For the open-state modification protocol, channels were held at −130 mV, given a 10-ms test pulse to −30 mV, and then exposed to MTSET for 50 ms at 0 mV. This process was repeated every 40 s with MTSET washout occurring at −130 mV. Test pulse current traces are plotted before and after each subsequent exposure to MTSET ( b , bottom). The brown line was included to highlight any changes in current amplitude. Peak sodium current does not decrease after exposure to MTSET while channels are closed or open, indicating that this mutant does not react with MTSET. Full size image Pore cysteine access is intracellularly gated If an intracellular gate exists within voltage-gated sodium channels, then we hypothesize that residues above the gate will be inaccessible to internally applied membrane impermeable MTSET while the gate is closed, but will become accessible when the gate is open. To test this prediction, we measured the accessibility of the introduced cysteine L1580C in Nav1.4-WSW channels to intracellularly applied MTSET in excised inside-out patches from Xenopus oocytes ( Fig. 2 ). On the basis of homology with bacterial sodium channel structures, L1580 is likely to line the pore above the putative gate at the S6 helix bundle crossing. To determine the state-dependent accessibility of L1580C, we estimated the rate of MTSET modification under conditions where we expect the channels to be predominantly either closed (−130 mV) or open (0 mV). For both cases, the extent of modification was assayed intermittently by examining the peak current response to a test pulse to −30 mV. 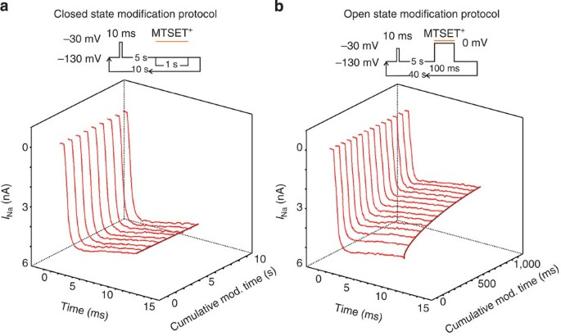Figure 2: State-dependent modification of L1580C. Closed-state (a, top) and open-state (b, top) modification protocols for monitoring modification by 200 μM MTSET applied to inside-out patches excised fromXenopusoocytes containing Nav1.4-WSW-L1580C channels. Test pulse current traces for closed-state modification (a, bottom) and open-state modification (b, bottom) are plotted before and after each subsequent exposure to MTSET. Peak sodium current does not change when MTSET is applied to closed channels; however, sodium current decreases after each 100 ms exposure of MTSET to open channels. Figure 2 shows that L1580C undergoes no apparent modification while the channel is closed, whereas MTSET application while the channel is held open results in a time-dependent decrease in current amplitude, indicating that this position is accessible in the open state. A cytoplasmic gate below L1580 could explain why this site is protected from MTSET while the channels are closed, but accessible while the channel is open. Figure 2: State-dependent modification of L1580C. Closed-state ( a , top) and open-state ( b , top) modification protocols for monitoring modification by 200 μM MTSET applied to inside-out patches excised from Xenopus oocytes containing Nav1.4-WSW-L1580C channels. Test pulse current traces for closed-state modification ( a , bottom) and open-state modification ( b , bottom) are plotted before and after each subsequent exposure to MTSET. Peak sodium current does not change when MTSET is applied to closed channels; however, sodium current decreases after each 100 ms exposure of MTSET to open channels. Full size image Channel gating determines MTSET accessibility If changes in accessibility between closed and open states reflect conformational changes that gate access to the pore, then the rates of modification should follow the relative probability of channel opening. We predict that changes in accessibility between closed and open states reflect conformational changes that gate access to the pore. Conversely, these changes could also result from changes in the membrane electric field even in absence of a conformational change [23] . In the latter case, we would expect that accessibility rates to vary linearly with voltage, whereas in the former case the voltage dependence of accessibility should correspond to the voltage dependence of pore opening. To test this, we measured the voltage dependence of MTSET accessibility to S1578C as well as tail currents from −130 to +30 mV. Similar to L1580C, S1578C is only accessible while channels are open but confers a greater degree of current inhibition on modification, which facilitates accessibility measurements. 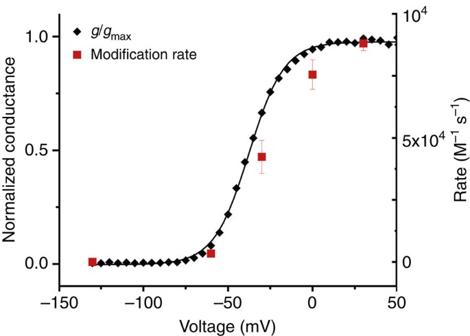Figure 3: Changes in accessibility follow channel gating. The rates of modification (red boxes) in the presence of MTSET perfused on inside-out patches held at different voltages during MTSET exposure are plotted alongside the conductance–voltage relation (black diamonds) for Nav1.4-WSW-L1578C channels. The red vertical error bars represent the s.d. of the modification rates (n=3); the solid black line is a Boltzmann function fit to the mean values for independent fits to three experiments. These data demonstrate that voltage-dependent changes in channel open probability and the rates of modification at different voltages are correlated. Figure 3 shows that the MTSET modification rates of S1578C are correlated with changes in channel open probability derived from macroscopic measurements. Therefore, changes in MTSET accessibility at sites in the S6 of domain IV track activation gating of sodium channels. Figure 3: Changes in accessibility follow channel gating. The rates of modification (red boxes) in the presence of MTSET perfused on inside-out patches held at different voltages during MTSET exposure are plotted alongside the conductance–voltage relation (black diamonds) for Nav1.4-WSW-L1578C channels. The red vertical error bars represent the s.d. of the modification rates ( n =3); the solid black line is a Boltzmann function fit to the mean values for independent fits to three experiments. These data demonstrate that voltage-dependent changes in channel open probability and the rates of modification at different voltages are correlated. Full size image C-terminal cysteine is not protected by a closed pore gate In contrast to the state-dependent accessibility of S1578C and L1580C, we expect that sites below the gate will be accessible to MTSET whether the channel is open or closed. On the basis of homology with prokaryotic sodium channel structures, F1594 appears to be located just below the S6 helix bundle crossing, and thus may not be protected from MTSET modification by gate closure. To test this, we measured MTSET accessibility rates for Nav1.4-WSW-F1594C channels in both closed and open states ( Fig. 4a,b ). Substantial modification occurs whether MTSET is applied to channels held at −130 mV or 0 mV, indicating that F1594C can react with intracellular reagents regardless of whether the channel is closed or open. This suggests that F1594 is located below the pore gate. 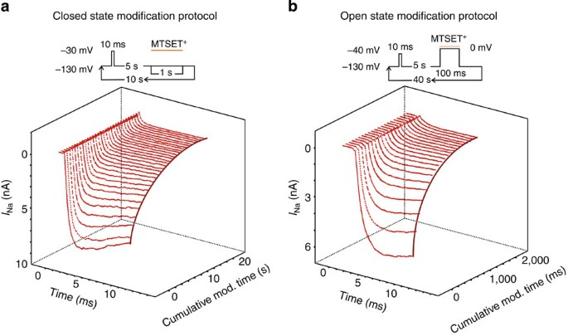Figure 4: Modification of F1594C. Closed-state (a, top) and open-state (b, top) modification protocols for monitoring modification by 100 μM MTSET applied to inside-out patches excised fromXenopusoocytes containing Nav1.4-WSW-F1594C channels. Test pulse current traces for closed-state modification (a, bottom) and open-state modification (b, bottom) are plotted before and after each subsequent exposure to MTSET. Peak sodium current decreases after each 100 ms exposure of MTSET to both closed and open channels. Figure 4: Modification of F1594C. Closed-state ( a , top) and open-state ( b , top) modification protocols for monitoring modification by 100 μM MTSET applied to inside-out patches excised from Xenopus oocytes containing Nav1.4-WSW-F1594C channels. Test pulse current traces for closed-state modification ( a , bottom) and open-state modification ( b , bottom) are plotted before and after each subsequent exposure to MTSET. Peak sodium current decreases after each 100 ms exposure of MTSET to both closed and open channels. Full size image Mapping accessibility of domain IV S6 residues Given that S1578C and F1594C are both accessible to MTSET while the channel is open, but only F1594C is accessible while the channel is closed, the pore gate must be located somewhere between S1578 and F1594. To determine the gate’s location, we systematically tested the accessibility of individual substituted cysteines along the DIV S6 from position 1578 to 1594. We define the position of the gate to be the site at which we first see significant closed-state accessibility. 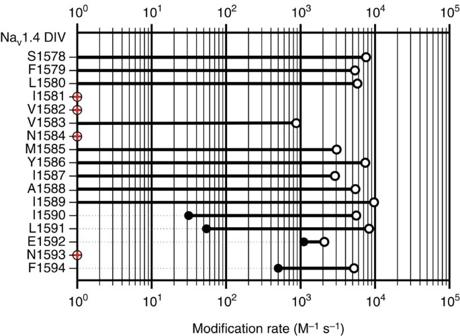Figure 5: State-dependent accessibility of DIV S6 cysteine mutants. Cysteine modification rates in the closed (filled circles) and open (open circles) states are plotted on a logarithmic scale for positions 1578-1594. Each point is the mean of three experiments. The length of the bar represents the fold change in rate between the closed and open states. Sites above I1590 have closed-state reactivity values <1 M−1s−1. I1581C, V1582C, N1584C and N1593C displayed no change in peak current after MTSET exposure (red marks). Depending on the rates of modification, the concentration of MTSET used to test each site ranged from 100 μM to 2 mM. Figure 5 shows the rates of MTSET modification in both closed and open states at each position. These data reveal a distinct delineation between sites exhibiting state-dependent and state-independent accessibility to MTSET. Sites above I1590 show modification rates less than 1 M −1 s −1 in the closed state, but these increase by more than 10,000-fold in the open state. The large increase in reactivity on channel opening implies that these sites are protected from MTSET modification while channels are closed, presumably by the gate. At or below position 1590, we see significant modification in both closed and open states. A more than 100-fold increase in closed-state accessibility at these sites indicates that these cysteines are no longer protected by the gate. The much smaller differences between the open- and closed-state modification rates might reflect conformational changes of this region associated with channel gating. Thus, much like the voltage-gated Shaker potassium and Cav2.1 channels, MTSET access to the pore of a voltage-gated sodium channel is regulated by an intracellular gate at or in the immediate vicinity of I1590 (refs 10 , 12 ). Figure 5: State-dependent accessibility of DIV S6 cysteine mutants. Cysteine modification rates in the closed (filled circles) and open (open circles) states are plotted on a logarithmic scale for positions 1578-1594. Each point is the mean of three experiments. The length of the bar represents the fold change in rate between the closed and open states. Sites above I1590 have closed-state reactivity values <1 M −1 s −1 . I1581C, V1582C, N1584C and N1593C displayed no change in peak current after MTSET exposure (red marks). Depending on the rates of modification, the concentration of MTSET used to test each site ranged from 100 μM to 2 mM. Full size image Conserved hydrophobic gate in canonical channels We aligned the pore sequences of the rat Kv1.2 and Shaker potassium channels with several bacterial voltage-gated sodium channels and the individual pore domains of rat Nav1.4 channels to assess the likelihood that (1) the location of the pore gate inferred from our accessibility studies represents a conserved feature among voltage-gated sodium channels and (2) our proposed gate in sodium channels is consistent with the gate inferred from similar accessibility studies in Shaker potassium and voltage-gated calcium channels ( Fig. 6a ). The multiple sequence alignment was performed using Expresso [24] , which utilizes the structural X-ray crystallographic data available for Kv1.2 (PDB 2A79) [7] , NavAb (PDB 4EKW) [25] , NavMs (PDB 4F4L) [16] and NavRh (PDB 4DXW) [26] . The reliability of the alignment at each position was judged by the CORE index score as reported by T-Coffee [27] . This score was maximized in the regions corresponding to the selectivity filter and our proposed gate location in Nav1.4, but became progressively less reliable in regions associated with loops between helices or those extending into the cytoplasm as expected for less well-ordered structures. 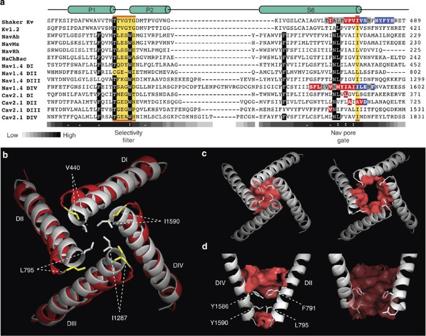Figure 6: Alignment of pore domains and homology models. (a) Aligned sequences of individual pore domains for rat Kv1.2, Shaker Kv, rat Nav1.4, rabbit Cav2.1 and the bacterial sodium channels NavAb, NavMs, NavRh and NaChBac (see Results). Red and blue highlighted residues in Nav1.4 DIV, Shaker Kv and Cav2.1 DI-III denote positions accessible to internal MTSET in both closed and open states (blue) or open states only (red). Residues highlighted in grey indicate positions where internal MTSET did not produce a functional change in the peak current response. Shaker Kv and Cav2.1 accessibility data are from previous experiments10,12. Residues aligned with those contributing to the selectivity filter and intracellular pore gate in Nav1.4 are highlighted in yellow. Highly conserved residues are shown on a black background. Grey scale bar below the sequences shows the CORE index reliability score at each position (light grey=low reliability, black=high reliability) along with an indicator for highly conserved (:) and semi-conserved (.) positions27. (b) Homology models of the pore lining S6 segments from each domain in rat Nav1.4 channels based on prokaryotic structures in either the closed pore (NavAb, white) or open pore (NavMs, red) conformations. View is from the cytoplasm looking up through the channel pore. The residues comprising the pore gate are shown in stick representation in both their closed (white) and open (yellow) configurations. Images were generated with PyMOL (The PyMOL Molecular Graphics System, Version 1.5.0.4; Schrödinger, LLC). (c) The solvent accessible surface at the gate region is shown in red for both the closed pore (left) and open pore (right) Nav1.4 models. View is the same as inb. (d) View of the gate region from within the plane of the membrane for closed (left) and open (right) Nav1.4 models. For clarity, only domains II and IV are shown. The residues contributing to the pore gate in the closed pore model are shown in stick representation and the solvent accessible surface is shown in red. For the open pore model, the solvent accessible surface is transparent so that the gate residues can be visualized. Figure 6: Alignment of pore domains and homology models. ( a ) Aligned sequences of individual pore domains for rat Kv1.2, Shaker Kv, rat Nav1.4, rabbit Cav2.1 and the bacterial sodium channels NavAb, NavMs, NavRh and NaChBac (see Results). Red and blue highlighted residues in Nav1.4 DIV, Shaker Kv and Cav2.1 DI-III denote positions accessible to internal MTSET in both closed and open states (blue) or open states only (red). Residues highlighted in grey indicate positions where internal MTSET did not produce a functional change in the peak current response. Shaker Kv and Cav2.1 accessibility data are from previous experiments [10] , [12] . Residues aligned with those contributing to the selectivity filter and intracellular pore gate in Nav1.4 are highlighted in yellow. Highly conserved residues are shown on a black background. Grey scale bar below the sequences shows the CORE index reliability score at each position (light grey=low reliability, black=high reliability) along with an indicator for highly conserved (:) and semi-conserved (.) positions [27] . ( b ) Homology models of the pore lining S6 segments from each domain in rat Nav1.4 channels based on prokaryotic structures in either the closed pore (NavAb, white) or open pore (NavMs, red) conformations. View is from the cytoplasm looking up through the channel pore. The residues comprising the pore gate are shown in stick representation in both their closed (white) and open (yellow) configurations. Images were generated with PyMOL (The PyMOL Molecular Graphics System, Version 1.5.0.4; Schrödinger, LLC). ( c ) The solvent accessible surface at the gate region is shown in red for both the closed pore (left) and open pore (right) Nav1.4 models. View is the same as in b . ( d ) View of the gate region from within the plane of the membrane for closed (left) and open (right) Nav1.4 models. For clarity, only domains II and IV are shown. The residues contributing to the pore gate in the closed pore model are shown in stick representation and the solvent accessible surface is shown in red. For the open pore model, the solvent accessible surface is transparent so that the gate residues can be visualized. Full size image We also aligned the pore sequences of several bacterial sodium channels with the individual pore domains in human Nav1.x ( x =1..9), Cav1.x ( x =1..4) and Kv1.x ( x =1..7) channels using Muscle [28] ( Supplementary Fig. 1 ). As described above, the reliability in the alignment was maximized in the region of our proposed gate in Nav1.4 DIV across channel types, isoforms and domains. Where comparable, the alignment in the vicinity of the gate was identical to that shown in Fig. 6a . Consistent with the reliability scores, multiple sequence alignments with several other programs including Clustal Omega [29] , T-Coffee [27] and TM-Coffee [30] resulted in identical alignments in our proposed gate region, differing only in the placement of the gaps in the surrounding regions of lower reliability. The residues aligned with the pair of isoleucines I1589 and I1590 in Nav1.4 DIV, between which we observe a striking change in state-dependent accessibility, are nearly uniformly composed of the hydrophobic residues I, V and L across Nav, Cav and Kv isoforms and domains ( Fig. 6a ; Supplementary Fig. 1 ). The only exceptions are for domains II and III in calcium channels where the aligned residues are IA and FV, respectively. The gate location in Shaker potassium channels agrees well with our observations in Nav1.4, with the change from state-dependent to state-independent accessibility for rat Nav1.4 DIV and Shaker Kv occurring within one position in their aligned pore sequences ( Fig. 6a ). Furthermore, positions immediately preceding those aligned with rat Nav1.4-I1589 are predominantly highly conserved hydrophobic residues with a few polar residues and no charged residues. In contrast, polar and charged residues are abundant following the hydrophobic stretch up to positions aligned with rat Nav1.4-I1590, as expected for a transition from a transmembrane helix to a cytoplasmic motif. Furthermore, accessibility studies in rabbit Cav2.1 channels indicate the presence of an intracellular gate within two residues of rat Nav1.4-I1590 in their aligned sequences ( Fig. 6a ) [12] . Taken together, these observations suggest that access to the pore in Nav1.4, Shaker Kv and Cav2.1 channels is similarly gated by hydrophobic residues at the intracellular end of the sixth transmembrane helices, and that this is a conserved feature amongst the founding members of the VGIC superfamily. A structural model of pore gating in sodium channels Given the strong sequence alignment in the proposed gate region, we posit that pore gating involves conserved structural features in prokaryotic and eukaryotic voltage-gated sodium channels. To explore this possibility, we generated homology models of S6 segments of Nav1.4 based on structures of prokaryotic sodium channels from Arcobacter butzleri (NavAb [8] ) and Magnetococcus sp. (NavMs [16] ; see Methods). Compared with the Kv channels, the bacterial sodium channels have a greater degree of homology to the eukaryotic sodium channels and, therefore, were the preferred templates for homology modelling. For instance, they lack the highly conserved PVP motif of Kv channels that would introduce a kink in the S6 helix. Our models for the pore of Nav1.4 show that the backbone of the S6 transmembrane helix overlaps nearly perfectly between closed and open conformations near its amino-terminal (extracellular) end, whereas the carboxy-terminal (intracellular) end of the helix is bent outwards away from the pore axis in the open pore model relative to that of the closed pore ( Fig. 6b ). Notably, the residues V440, L795, I1287 and I1590 from aligned positions in each of the four domains face in towards the pore axis in the closed pore model where they come within close proximity and appear to form a hydrophobic barrier that could occlude the pore. In the open pore model, these residues are moved radially outwards away from the pore axis and are no longer in close proximity. To determine whether our models for Nav1.4 are reflective of actual closed and open pore conformations, we computed the solvent accessible surface through the pore formed by the intracellular ends of the S6 pore helices in each domain using HOLLOW with a grid spacing of 0.2 Å (ref. 31 ). Figure 6c,d illustrates the inability of water to traverse the closed pore, which is occluded by a hydrophobic gating ring comprising V440, L795, I1287 and I1590, whereas an aqueous channel is formed on the dispersion of this gating ring in the open pore model. Interestingly, our homology models of the closed state suggest that another set of conserved hydrophobic residues, one helical turn above the gating ring, may come together and stabilize the closed gate. The exact role of these residues will need to be elucidated in future experiments. Using a fast inactivation-deficient sodium channel, we have shown that cysteine residues inserted into the pore lining DIV S6 helix react in a state-dependent manner with intracellular MTSET. At positions 1578-1594, we observe no change in current amplitude after MTSET is applied to closed channels, consistent with the notion that these sites are not accessible in the closed state. In contrast, we observe a >10,000-fold increase in accessibility at these same sites when channels are held open. Cysteine residues below these positions (1590–1594) are accessible to modification by MTSET regardless of whether the channel is closed or open. Our observations suggest that activation gating in voltage-gated sodium channels involves the rearrangement of a discrete structural feature located near the membrane/cytoplasm interface that physically occludes the pore. Our homology model, as well as the computed changes in the solvent accessible surface of the closed and open pore, is consistent with this conclusion. However, we cannot determine whether gating is a consequence of DIV S6 motion or that of neighbouring helices. Our study provides information only about the location of the pore gate but not about the dynamics or motions of the gate. Previous attempts to determine the location of the gate in eukaryotic voltage-gated sodium channels were not productive in large part because of the presence of fast inactivation in wild-type channels. MTS accessibility measurements of introduced cysteines in the S6 showed that only two out of the 17 sites tested showed substantial current inhibition on modification [19] . Moreover, these two sites only became accessible on high frequency stimulation and their modification rates were at least 1,000-fold lower than the open-state modification rates in Shaker potassium channel [10] . Another study based on mutational analysis suggested that a group of conserved aromatic residues near the cytoplasmic end of each S6 helix from Nav1.7 forms a hydrophobic plug that acts as a gate [32] . Substitutions of less bulky amino acids in those positions were found to destabilize the closed state relative to the open state. However, this does not rule out the possibility that the mutations indirectly affect the stability of the gate. Not surprisingly, their placement of the gate is not consistent with our data in that the activation gate determined by accessibility measurements is more than one helical turn above their site. Accessibility studies have been performed on several members within the VGIC superfamily, but it is unclear whether these functional data are compatible with structural data, as few structures are available for comparison in both closed and open states. Modification data have been obtained for the Shaker potassium channel; however, all the structures of the Kv channels are of the open state [7] , [33] . Without a picture of the closed channel, it is difficult to specifically define the molecular identity of the gate. Recently, structures of bacterial sodium channels have been solved in different states [8] , [16] , [25] . Given the high degree of similarity between the S6 region of the eukaryotic and prokaryotic sodium channels, we were able to map functional data onto the structures by generating homology models. Structural analysis of our open- and closed-state models shows that when the channel is closed, a ring of four bulky hydrophobic residues create a narrow constriction (~3.8 Å). Hydrated Na + ions (~7.8 Å diameter) and MTSET (~5.8 Å headgroup diameter) will clearly not be granted passage through this gap. After channel activation, members of this ring move >2 Å away from the central axis of the pore. The pore is now >8 Å in diameter, which is sufficiently large to provide hydrated Na + ions and MTSET access to the pore. Strikingly, our accessibility measurements show that I1590 is the first residue to be modified even when channels are closed consistent with this being the barrier for ion conduction in the structural models. Structures of the prokaryotic sodium channel in the closed state show that the passage for ions becomes narrower further down the S6 helix, which led Shaya et al. [18] to suggest that the gate location is one helical turn below the hydrophobic residue identified in the present study. It is possible that bacterial sodium channels have additional barriers for ion conduction but those regions are not evolutionary conserved ( Fig. 6a ). They are replaced by aromatic residues in the eukaryotic sodium channels and, more importantly, these residues remain accessible to polar thiol reagents in the closed state. Sequence comparison shows that canonical voltage-gated ion channels, which include the voltage-gated sodium, potassium and calcium channels, all contain a three-residue hydrophobic stretch (hydrophobic triplet) followed by polar and charged residues ( Supplementary Fig. 2 ). This stretch is composed of the branched amino acids I, V and L. The transition from state-dependent to state-independent accessibility of Nav1.4 DIV occurs within one residue for that of the Shaker Kv channel and two for Cav2.1 channels, all of which are in the conserved hydrophobic stretch. Although DII and DIII of Cav1.x contain an alanine and a phenylalanine, respectively, in this stretch, we suspect that this does not significantly affect activation gating because only 2 of 12 residues are altered and they remain hydrophobic. In contrast, this hydrophobic triplet is disrupted in both CNG and BK channels by insertion of either multiple polar or negatively charged residues. Accessibility studies of both these channels have conclusively established that this region of the pore does not serve as the activation gate [5] , [13] , [14] . Given these differences between the intracellularly and non-intracellularly gated channels, we posit that this hydrophobic stretch is a key determinant of pore gating in canonical voltage-dependent ion channels. In conclusion, we provide a model for pore gating in sodium channels based on MTSET accessibility data and analysis of the closed and putatively open-state crystal structures of bacterial sodium channels. Given the remarkable agreement between functional data from eukaryotic channels and the structures of prokaryotic channels, our study suggests that the bacterial sodium channels may serve as excellent candidates for understanding some features of the gating process in eukaryotic sodium channels. Molecular biology and electrophysiology WSW was generated by Quikchange mutagenesis (Stratagene, CA) using WCW template DNA and subcloned into domain I of Na v 1.4 using Mfe I and BsiWI (C437S forward primer: 5′-CAACTGGATCTCCTGGGTGGTGGCCATGGCG-3′; C437S reverse primer: 5′-GGCCACCACCCAGGAGATCCAGTTGATGAGG-3′). Single cysteines 1,592–1,594 were created using Quikchange mutagenesis, confirmed by gene sequencing, and were then subcloned into domain IV of the WSW background using Xba I and BspEI (E1592C forward primer: 5′-CCTGTGCAATTTCAACGTGGCC-3′; E1592C reverse primer: 5′-CGTTGAAATTGCACAGGATGATAGC-3′; N1593C forward primer: 5′-CCTGGAGTGCTTCAACGTGGCC-3′; N1593C reverse primer: 5′-CGTTGAAGCACTCCAGGATGATAGC-3′; F1594C forward primer: 5′-GGAGAATTGCAACGTGGCCACCGAAG-3′; F1594C reverse primer: 5′-CACGTTGCAATTCTCCAGGATGATAGC-3′). Using the same restriction enzymes, individual cysteine residues 1578-1594 received from Drs Dorothy Hanck and John Kyle were subcloned into the WSW background. For expression, constructs were linearized by Not I digestion and transcribed in vitro using the T7 RNA polymerase kit (Ambion Inc., CA). α-subunit and β 1 -subunit cRNA were co-injected into defolliculated Xenopus laevis oocytes in a 1:1 ratio of 2 μg μl −1 α-subunit and 400 ng μl −1 β 1 subunit. Ionic currents were measured from inside-out patches excised from oocytes 3–6 days after injection. Standard solutions contained, in mM: NaF 100, KCl 20, EGTA 2, HEPES 10, MgCl 2 2.5, at pH 7.2 (bath); NaCl 115, KCl 5, CaCl 2 2, HEPES 10, at pH 7.2 (pipette). Typical pipette resistances were 500 kΩ–1.5 MΩ. On inside-out patch excision, currents were allowed to stabilize at −130 mV for 5 min. The voltage at which the conductance was half-maximal ( V 1/2 ) for the mutants tested in this study was in the range of −45 mV to −10 mV. On the basis of these values, the potentials for MTSET exposure was adjusted such that the open probabilities were close to maximum. For instance, I1590 has a V 1/2 value of −10 mV; therefore, its open state accessibility was checked at +20 mV. Chemical modification A stock solution of ~5 mM MTSET (Toronto Research Chemicals, Ontario) was prepared daily and kept on ice. This stock solution was diluted to 100 μM in bath solution and used immediately (within 1 min). Inside-out patches containing mutant channels were exposed to MTSET via a rapid perfusion system in which a computer-controlled valve was used to switch between standard bath solution and one containing MTSET [34] , [35] . By switching between our standard bath solution and one of a lower ionic strength, it is possible to assess the dead time of the perfusion apparatus (typically 150 ms). This time was determined for each set of experiments and was accounted for in order to synchronize it with voltage pulses that open and close the channel. This method ensures that the reported reaction rates take into account only at the time during which MTSET was present. Typical closed- and open-state modification protocols are described in Fig. 1 . For each experiment, the time constant of MTSET modification was calculated by plotting the cumulative exposure time to MTSET versus peak sodium current. The accessibility, or the apparent second-order rate constants, of MTSET to each cysteine mutant was determined by dividing the reciprocal of the time constant by the concentration of MTSET. After prolonged depolarizations, it has been observed that fast inactivation-deficient preparations of sodium channels display an increased propensity to enter into a slow-inactivated state [21] . This trend was also noticeable for each mutant used in our experiments. To make sure that test pulse sodium currents represent decay owing to MTSET modification and not forms of slow inactivation, we used mock open-state protocols in which bath solution and not MTSET was applied to determine the necessary time between each exposure sweep. This guaranteed that each successive test pulse reported inhibition of current owing to MTSET modification and not slow inactivation. Homology models The closed pore model template was generated by aligning two copies of the NavAb dimer structure (PDB 3RVY) to each of two subsequent domains in the NavMs tetramer (PDB 4F4L). The alignment consisted of minimizing the root mean squared deviation (r.m.s.d.) between backbone and C α atoms from the S5 helix through the selectivity filter and into the N-terminal half of the S6 helix (G129–V205 in NavAb, G130–T206 in NavMs) in Visual Molecular Dynamics [36] . These regions overlap well with an r.m.s.d.<0.42 Å for the aligned atoms. The C-terminal half of the S6 helix was excluded from the alignment as this region shows structural differences between NavAb and NavMs presumably due to the different conformation of the pore. The open pore model template was generated by similarly aligning the most bent pore domain in the NavMs structure (chain A) with each of the other three domains in NavMs (r.m.s.d.<0.12 Å for aligned atoms). Homology models based on the closed- and open-template structures described above were generated from the aligned sequences of each of the four domains in Nav1.4 with either NavAb or NavMs, as shown in Fig. 6a using the default options in Modeller [37] . In each case, 100 potential models were generated and both examined visually and ranked according to their Discrete Optimized Protein Energy (DOPE) score as assigned by Modeller. The position of the gate residues V440, L795, I1287 and I1590 showed little variation between potential closed pore models (C α r.m.s.d.<0.7 Å), with C α -C α distances between non-adjacent gate residues ranging from 9.7 to 11.6 Å. The hydrophobic residues I436, F791, F1283 and Y1586 one helical turn above the gate residues inferred from our accessibility studies adopted orientations in the closed pore models such that either all three aromatic residues were oriented towards the pore axis (group I), or two of the three aromatic residues were oriented towards the pore axis with the third being rotated upward towards the extracellular side of the membrane (group II). As the orientation of these aromatic side chains are not well constrained by the template structures (see Results), we arbitrarily selected a model from group I with the best score (ranked 6 out of 100 overall). Our observation that the pore gate may consist of two rings of hydrophobic residues based on the solvent accessible surface in the closed pore model does not rely on this choice, as a similar profile of solvent accessibility was obtained for the group II model having the best score. For the open pore structures, the position of the gate residues V440, L795, I1287 and I1590 was slightly more variable than for the closed pore models (C α r.m.s.d.<3.1 Å), with C α -C α distances between non-adjacent gate residues ranging from 14.2 to 22.9 Å. There was no obvious clustering of orientations for the aromatic side chains’ one helical turn above in the open pore models as was observed in the closed pore model candidates. Thus, we simply selected one of the top-ranked open pore models for which the three aromatics F791, F1283 and Y1586 were consistent with group II as described above (selected model ranked 17 out of 100 overall). For the final selected models, the C α -C α distance between non-adjacent gate residues V440, L795, I1287 and I1590 was ≤11.2 Å in the closed pore model and ≥16.7 Å in the open pore model. How to cite this article: Oelstrom, K. et al. Evolutionarily conserved intracellular gate of voltage-dependent sodium channels. Nat. Commun. 5:3420 doi: 10.1038/ncomms4420 (2014).